ID4 controls mammary stem cells and marks breast cancers with a stem cell-like phenotype Basal-like breast cancer (BLBC) is a heterogeneous disease with poor prognosis; however, its cellular origins and aetiology are poorly understood. In this study, we show that inhibitor of differentiation 4 (ID4) is a key regulator of mammary stem cell self-renewal and marks a subset of BLBC with a putative mammary basal cell of origin. Using an ID4GFP knock-in reporter mouse and single-cell transcriptomics, we show that ID4 marks a stem cell-enriched subset of the mammary basal cell population. ID4 maintains the mammary stem cell pool by suppressing key factors required for luminal differentiation. Furthermore, ID4 is specifically expressed by a subset of human BLBC that possess a very poor prognosis and a transcriptional signature similar to a mammary stem cell. These studies identify ID4 as a mammary stem cell regulator, deconvolute the heterogeneity of BLBC and link a subset of mammary stem cells to the aetiology of BLBC. The mammary gland offers a unique model for the study of epithelial stem cell biology and differentiation pathways since the majority of its development occurs after birth. At birth the mammary gland is composed of only a rudimentary ductal epithelial structure, and then fully develops during puberty and pregnancy [1] . The mature virgin mammary gland is composed of a bilayered ductal structure, comprised of two main terminally differentiated cell types, the inner luminal cell layer surrounded by a myoepithelial cell layer. Within the mammary epithelium there are marked proliferative bursts at puberty and during pregnancy requiring an increase in the stem/progenitor cell pool followed by rapid cell proliferation and differentiation. During pubertal development the terminal end buds (TEBs) are sites of massive tissue remodelling and are enriched for stem cell activity [2] , [3] . Investigation of the molecular mechanisms controlling mammary epithelial lineage commitment has led to the elaboration of a network of transcriptional pathways promoting luminal fate specification and terminal differentiation. Some of the earliest cell fate decisions within the mammary epithelial stem cell may be controlled by the Notch and Hedgehog pathways to promote luminal differentiation [4] , [5] . The subsequent activation of transcription factors GATA-binding protein 3 (Gata3), breast cancer type-1 susceptibility protein (Brca1), E74-like factor 5 Elf-5 (Elf5) and Forkhead box protein M1 (FoxM1) and Notch signalling are required for luminal progenitor cell fate and then terminal ductal/alveolar luminal cell differentiation [6] , [7] , [8] , [9] , [10] . In contrast, the transcriptional regulators of stem cell maintenance and myoepithelial cell differentiation are poorly described, in part due to the difficulties in purifying stem cells from myoepithelial cells for transcriptional and biochemical characterization [11] , [12] . On the basis of expression of cell surface antigens CD24 and CD29 or CD49f [13] , [14] , stem cells capable of reconstituting mammary glands in vivo can only be isolated to a purity of ~1–5%, the remainder comprising myoepithelial cells. It is established that Wnt signalling is necessary for mammary stem cell (MaSC) maintenance [11] , and that the expression of transcription factors Slug and Sox9 is sufficient to reprogramme the stem cell state from luminal epithelial cells [15] . Transcriptional profiling of the mixed ‘basal cell’ population reveals specific expression of many genes compared with luminal progenitors or committed luminal cells, with the helix-loop-helix (HLH) transcription factor inhibitor of differentiation 4 (ID4), one of the highest among these genes in both the human and murine basal population [16] . Id proteins regulate stem cell homeostasis and fate commitment in various cell types, including neuronal [17] , hematopoietic [18] , [19] and embryonic [20] cells. The role of the Id proteins has been studied to a limited extent in mammary gland development. Id1 is unnecessary for mammary gland development [21] , whereas Id2 is necessary for normal RANK signalling within the mammary gland [22] . Id4 loss leads to a delay in pubertal mammary gland development, associated with an increase in p38MAPK phosphorylation; however, this study did not identify a direct molecular link between Id4 as a transcriptional regulator and changes in p38MAPK phosphorylation nor did it address the role of Id4 in mammary epithelial fate decisions [23] . Studies of mammary development have led to great insights into breast cancer biology, and it is now clear that a number of transcription factors controlling luminal lineage commitment, such as Gata3 and Brca1 , are potent breast tumour suppressors, frequently mutated in malignancy [6] , [7] , [10] , [24] . Breast cancer is a heterogeneous disease, with at least five major subtypes distinguished by unique clinical behaviour, molecular signatures, genomic features and histopathology [25] . The basal-like breast cancer (BLBC) subtype comprises ~18% of all breast cancer diagnoses and is associated with early age of diagnosis, high grade and early relapse [26] , [27] . Considerable heterogeneity in gene expression and clinical prognosis exists within the BLBC subtype, where ~30–50% of patients relapse within 3–5 years while the remaining patients have good long-term survival (reviewed in ref. 28 ). Thus markers that can stratify survival in this subtype of breast cancer are of particular clinical significance. There is increasing evidence that the different subtypes of breast cancer are derived from different cells of origin within the stem cell hierarchy. Due to the frequent expression of basal cytokeratins by BLBC, the cell of origin for BLBC was initially thought to be a basal stem or myoepithelial cell. More recent molecular profiling of BLBC suggests luminal progenitors as the cell of origin for BLBCs in BRCA1 mutation carriers [29] , [30] , although the generality of this finding across the diversity of sporadic BLBC is not yet clear. In this study, we provide evidence that ID4 is a key controller of mammary stem/progenitor cell self-renewal, acting upstream of Notch signalling to repress luminal fate commitment. ID4 is overexpressed and required by a subset of BLBCs, and patients with ID4 + BLBCs have particularly poor prognosis and a stem-like transcriptional profile. Id4 expression is enriched in MaSCs We detected Id4 immunoreactivity within the nuclei of the basal cell layer of mammary glands, including the cap cells and some body cells of the TEBs of the pubertal gland ( Supplementary Fig. 1a ). Co-immunofluorescence demonstrated that Id4 co-localized with the basal cell marker p63 but not with the luminal cell marker cytokeratin 8 (CK8) ( Supplementary Fig. 1b ). Basal cells in the duct showed heterogeneous expression of Id4 ( Supplementary Fig. 1b ), with particularly high expression, when compared with ductal basal cells, in the cap cells of TEBs of pubertal mice ( Fig. 1a ), a location previously reported to be enriched for mammary stem and progenitor cells [2] , [3] . The exclusive expression of Id4 within the basal cell population was confirmed using adult mice heterozygous for an enhanced green fluorescent protein (EGFP) allele knocked into the Id4 locus, which have previously been used to show an important role for Id4 in neural stem cell maintenance [31] . EGFP expression was analysed in the mammary epithelial basal (CD24 + , CD29 hi and CD61 + ), luminal progenitor (CD24 + ,CD29 lo and CD61 + ) and mature luminal (CD24 + , CD29 lo and CD61 − ) subpopulations by flow cytometry [6] . EGFP expression was restricted to the basal compartment, where ~16% of basal cells highly expressed EGFP ( Fig. 1b ). To determine whether Id4 hi cells within the basal compartment were enriched for stem cell activity, we transplanted CD29 hi EGFP hi and CD29 hi EGFP lo basal cells at two doses (100 and 500 cells) into the contralateral glands of 3-week-old FVB/N mice that had undergone surgical clearing of endogenous mammary epithelium. After 8 weeks, EGFP hi cells had engrafted to form mammary ductal trees at a significantly greater frequency at both cell doses, with an overall sevenfold increase in the proportion of mammary repopulating units (MRUs) in the Id4 EGFP hi cells than the Id4 EGFP lo cells ( P =0.005) ( Fig. 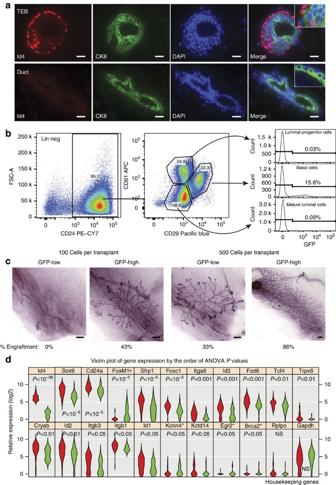Figure 1: Identification and functional characterization of Id4-positive MECs. (a) Id4 and cytokeratin 8 (CK8) expression detected by immunofluorescence in terminal end buds (upper panels) and mature ducts (lower panels) of 8-week-old wild-type mice. Scale bars, 20 μm. Representative image from five animals analysed. (b) Id4GFP reporter activity in MEC subsets identified by CD24, CD29 and CD61 immunostaining and flow cytometry. Representative histograms from five independent experiments. (c) Sorted CD29hi/GFPhiand CD29hi/GFPlomammary epithelium from Id4GFP/+mice were transplanted at two doses (100 and 500 cells) into the cleared mammary fat pad of naive FVB/N mice (seven glands per group) and analysed by whole-mount histology 8 weeks later. Percentage of transplanted mammary glands that showed a positive engraftment indicated below. Scale bars, 1 mm. (d) Single-cell RT–PCR for Id4 and MEC differentiation markers in Id4hi(top quartile; red) and Id4lo(bottom quartile; green) cells. All genes with significantly altered expression are shown withPvalue (ANOVA). * Indicates a negative correlation. 1c ; Supplementary Table 1 ). Figure 1: Identification and functional characterization of Id4-positive MECs. ( a ) Id4 and cytokeratin 8 (CK8) expression detected by immunofluorescence in terminal end buds (upper panels) and mature ducts (lower panels) of 8-week-old wild-type mice. Scale bars, 20 μm. Representative image from five animals analysed. ( b ) Id4GFP reporter activity in MEC subsets identified by CD24, CD29 and CD61 immunostaining and flow cytometry. Representative histograms from five independent experiments. ( c ) Sorted CD29 hi /GFP hi and CD29 hi /GFP lo mammary epithelium from Id4 GFP/+ mice were transplanted at two doses (100 and 500 cells) into the cleared mammary fat pad of naive FVB/N mice (seven glands per group) and analysed by whole-mount histology 8 weeks later. Percentage of transplanted mammary glands that showed a positive engraftment indicated below. Scale bars, 1 mm. ( d ) Single-cell RT–PCR for Id4 and MEC differentiation markers in Id4 hi (top quartile; red) and Id4 lo (bottom quartile; green) cells. All genes with significantly altered expression are shown with P value (ANOVA). * Indicates a negative correlation. Full size image To further explore the biology of Id4 hi basal cells at a cellular level, we used the murine mammary Comma-D cell line model that has been used previously to analyse mammary stem and progenitor cells [32] , [33] , [34] . When transplanted into the cleared fat pads of syngenic BALB/c mice, Comma-D cells formed relatively normal mammary outgrowths composed of bilayered ducts with Id4-positive basal cells and Id4-negative luminal cells ( Supplementary Fig. 1c,d ), suggesting a functional mammary epithelial lineage hierarchy exists within these cells. When cultured in vitro , Comma-D cells maintain a heterogeneous mixture of cells with basal and luminal features, including cells with diverse expression of Id4 as observed in vivo ( Supplementary Fig. 1e ). We used single-cell multiplexed reverse transcriptase (RT)–PCR to study the gene expression of unsorted Comma-D cells to gain an insight into whether Id4 hi cells possessed a MaSC signature. Using integrated microfluidic chambers, 166 individual Comma-D cells were analysed for expression of 92 genes of interest and 3 housekeeping genes. Selected genes included markers of mammary basal, progenitor and differentiated cells [13] , [14] , [35] , [36] , and common epithelial markers ( Supplementary Data 1 ). Confirming our observation by immunofluorescence (IF) ( Supplementary Fig. 1e ), Id4 messenger RNA (mRNA) was also heterogeneously expressed, while housekeeping genes were consistently expressed by all cells ( Supplementary Fig. 2 ). Unsupervised clustering showed that Id4 associated with the expression of other Id proteins and markers of stem and basal cells such as Sox9 ( Supplementary Fig. 2 ). To determine the genes with which Id4 was statistically significantly associated, gene expression of the top and bottom quartile Id4-expressing cells was analysed and visualized using violin plots ( Fig. 1d ) or using box plots ( Supplementary Fig. 3 ). Id4 expression was significantly correlated with high expression of the canonical basal and MaSC markers Itgα6 (CD49f [13] ) and Itgb1 (CD29; ref. 14 ) and with other Id family members Id1, Id2 and Id3. Id4 expression also positively correlated with 7 of 22 markers of fetal MaSC (fMASC) morphogenesis (CD24a, Sfrp1, Foxc1, Fzd6, Trpv6, Cryab and Kctd14) ( Fig. 1d ), previously shown to be elevated in poor prognosis BLBC [36] . In contrast, Id4 was not associated with any of the seven markers of luminal differentiation analysed, such as the oestrogen receptor and Gata3. The gene most robustly positively associated with Id4 expression was Sox9 (approximately fourfold higher in Id4 + cells; P <10 −5 ), a master regulatory transcription factor required and sufficient for MaSC activity [15] . In contrast, Id4 was strongly negatively correlated with FoxM1 (~15-fold lower in Id4 + cell; P <10 −5 ), a transcriptional repressor highly expressed in, and required by, luminal progenitors [10] . Together, these results demonstrate that Id4 expression is localized to regions of stem cell activity, that cells expressing Id4 are enriched for stem cell activity and that there is a stem-like gene expression programme in Id4 hi cells with similarities to adult and fetal stem cell signatures. Id4 is required for mammary ductal morphogenesis To further understand Id4’s functional role in mammary development, we examined ductal elongation and ductal morphogenesis in the mammary glands of 8-week-old adult Id4 −/− mice. Wholemount histology showed that Id4 −/− glands were poorly developed, with a fourfold reduction in the area of fat pad filled at 8 weeks of age ( Fig. 2a ). These results confirm the findings of Dong et al . [23] that Id4 is critical for ductal elongation. To determine whether this phenotype was caused by a cell-autonomous stem cell defect, we transplanted Id4 −/− mammary epithelial cells (MECs) into the cleared mammary fat pad of wild-type recipients at limiting dilutions. These experiments revealed a reduction in the frequency of MRUs in Id4 −/− mammary glands compared with controls with a 46% reduction in the frequency of MRUs in the Id4 −/− glands ( P =0.025) ( Table 1 ). Furthermore, in glands where engraftment did occur, there was a ~50% reduction in the extent of ductal invasion ( Fig. 2b ). Interestingly, there was no reduction in the proportion of total basal cells in the Id4 −/− glands when compared by flow cytometry ( Supplementary Fig. 4a,b ). This may be due to compensatory upregulation of Id1 and Id3 in the Id4 null glands ( Supplementary Fig. 4c ). To further validate the necessity of a cell intrinsic role for Id4 in epithelial homeostasis, we analysed Id4 knockdown by two independent short hairpin RNA (shRNA) in Comma-D cells ( Fig. 2c ); these led to a significant inhibition of proliferation in vitro ( P <0.0002, two-way analysis of variance (ANOVA), n =3) ( Fig. 2d ). 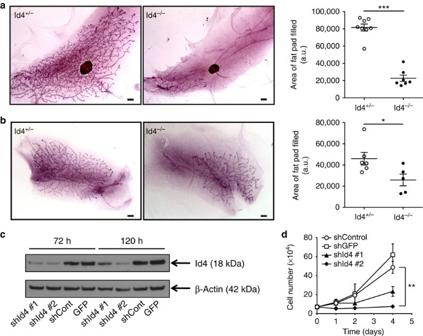Figure 2: Impact of Id4 deficiency on ductal morphogenesis and proliferation. (a) Whole-mount staining of Id4+/−and Id4+/+mammary glands at 8 weeks of age. Graphs indicate the mean±s.e.m. Id4+/−n=8, Id4−/−n=7. ***P<0.0005, unpairedt-test. Scale bars, 1 mm. (b) Analysis of the ability of epithelium from Id4−/−and Id4+/−mice to fill a mammary fat pad. Graphs indicate the mean±s.e.m. Id4+/−n=6, Id4−/−n=5. *P<0.05, unpairedt-test. Scale bars, 1 mm. (c) Western blot following Id4 knockdown by two independent shRNA (shId4 #1 and shId4 #2) compared with a scrambled control (shCont) and GFP-transduced Comma-D cells (for full western blot seeSupplementary Fig. 9). (d) Proliferation assays by cell counting following Id4 knockdown using two independent shRNA constructs and two independent controls (shControl and shGFP). (n=3 independent experiments) **P<0.0002, two-way ANOVA. Figure 2: Impact of Id4 deficiency on ductal morphogenesis and proliferation. ( a ) Whole-mount staining of Id4 +/− and Id4 +/+ mammary glands at 8 weeks of age. Graphs indicate the mean±s.e.m. Id4 +/− n =8, Id4 −/− n =7. *** P <0.0005, unpaired t -test. Scale bars, 1 mm. ( b ) Analysis of the ability of epithelium from Id4 −/− and Id4 +/− mice to fill a mammary fat pad. Graphs indicate the mean±s.e.m. Id4 +/− n =6, Id4 −/− n =5. * P <0.05, unpaired t -test. Scale bars, 1 mm. ( c ) Western blot following Id4 knockdown by two independent shRNA (shId4 #1 and shId4 #2) compared with a scrambled control (shCont) and GFP-transduced Comma-D cells (for full western blot see Supplementary Fig. 9 ). ( d ) Proliferation assays by cell counting following Id4 knockdown using two independent shRNA constructs and two independent controls (shControl and shGFP). ( n =3 independent experiments) ** P <0.0002, two-way ANOVA. Full size image Table 1 Limiting dilution analysis of the mammary repopulating frequency of unsorted mammary epithelial cells from Id4 +/− and Id4 −/− mice. Full size table Id4 is a key controller of luminal differentiation pathways Given that Id4 was highly expressed in mammary basal cells yet undetectable in luminal epithelium ( Fig. 1b ) and that Id4 expression was required for normal MaSC activity, we asked whether Id4 was sufficient to prevent luminal differentiation of mammary epithelial stem cells. The Comma-D cell line model undergoes luminal differentiation over a 4-day time course of confluence and growth factor withdrawal. Overexpression of Id4 did not alter proliferation of Comma-D cells in this assay ( Supplementary Fig. 5a ), but did upregulate constitutive cytokeratin 14 expression and markedly inhibited terminal luminal cell differentiation as measured by milk protein production and CK8 expression ( Supplementary Fig. 5b,c ). The inhibition of milk protein production by Id4 overexpression confirm the findings of Shan et al . [37] in the related HC11 cell line. To determine the mechanism by which Id4 controls luminal commitment of MaSCs, we examined expression of Brca1, Elf5 and activation of the Notch pathway, all of which are required for appropriate luminal epithelial commitment by MaSCs [5] , [8] , [9] . Id4 overexpression reduced constitutive expression of the luminal progenitor marker Brca1 ( Fig. 3a ). Under differentiation conditions, Comma-D cells upregulate Elf5 expression and Notch signalling as measured by an approximately ninefold increase in expression of the Notch target gene Hey1, and these increases were markedly inhibited by Id4 overexpression ( Fig. 3a ). In addition, gene expression analysis of Id4 −/− mammary glands revealed a marked increase in the expression of Notch pathway genes Hey1 , Notch1 and Jag1 ( Fig. 3b ), consistent with a role for Id4 in suppressing Notch pathway activity. 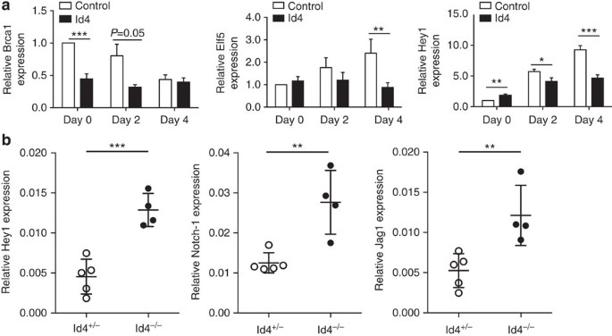Figure 3: Regulation of pathways controlling luminal fate commitment by Id4. (a) mRNA expression of Brca1 (n=5/group), Elf5 (n=7/group) and Hey1 (n=7/group) in Comma-D cells over a time course of luminal differentiation in cells overexpressing Id4 or a control. Graphs represent the mean±s.e.m. (b) mRNA expression of Notch pathway components Hey1, Notch1 and Jag1 in mammary glands from 8-week-old Id4−/−mice (n=4) compared with controls (n=5). Graphs represent the mean±s.e.m. *P<0.05, **P<0.01, ***P<0.001, unpairedt-test. Figure 3: Regulation of pathways controlling luminal fate commitment by Id4. ( a ) mRNA expression of Brca1 ( n =5/group), Elf5 ( n =7/group) and Hey1 ( n =7/group) in Comma-D cells over a time course of luminal differentiation in cells overexpressing Id4 or a control. Graphs represent the mean±s.e.m. ( b ) mRNA expression of Notch pathway components Hey1, Notch1 and Jag1 in mammary glands from 8-week-old Id4 −/− mice ( n =4) compared with controls ( n =5). Graphs represent the mean±s.e.m. * P <0.05, ** P <0.01, *** P <0.001, unpaired t -test. Full size image To test whether the observed reduction in Notch signalling was sufficient to account for the inhibition of luminal differentiation by Id4 overexpression, we treated Comma-D cells with DAPT (N-[N-(3,5-Difluorophenacetyl)-L-alanyl]-S-phenylglycine t-butyl ester), a gamma-secretase inhibitor that prevents Notch receptor cleavage and activation [38] . DAPT treatment phenocopied Id4 overexpression by suppressing the induction of Hey1, cytokeratin 8 and Elf5 expression through the time course of in vitro differentiation ( Fig. 4a,b ). Unlike Id4 overexpression, DAPT treatment did not inhibit expression of Brca1 ( Fig. 4c ) and only partially suppressed β-casein expression when compared with Id4 overexpression ( Fig. 4c versus Supplementary Fig. 5c ). Id4 was previously suggested to regulate mammary epithelial proliferation through suppression of p38MAPK activity, as determined by p38MAPK phosphorylation [23] . However, overexpression of Id4 in Comma-D cells did not suppress, nor did Id4 knockdown enhance, the expression of total or phospho-p38MAPK ( Supplementary Fig. 6 ). 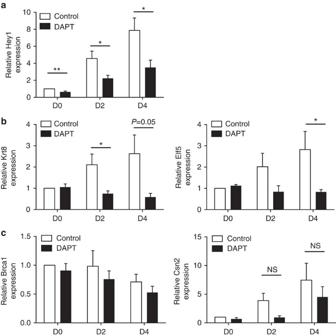Figure 4: Expression of differentiation markers following pharmacological Notch pathway inhibition. (a) Expression of notch target gene Hey1 in Comma-D cells treated with the notch inhibitor DAPT over a time course of confluence. (b) Luminal differentiation as measured by Krt8 and Elf5 expression following DAPT treatment. (c) Impact of DAPT treatment on Brca1 and Csn2 expression in Comma-D cells. Graphs represent the mean±s.e.m. *P<0.05, **P<0.01, NS=not significant, unpairedt-test.n=5. Figure 4: Expression of differentiation markers following pharmacological Notch pathway inhibition. ( a ) Expression of notch target gene Hey1 in Comma-D cells treated with the notch inhibitor DAPT over a time course of confluence. ( b ) Luminal differentiation as measured by Krt8 and Elf5 expression following DAPT treatment. ( c ) Impact of DAPT treatment on Brca1 and Csn2 expression in Comma-D cells. Graphs represent the mean±s.e.m. * P <0.05, ** P <0.01, NS=not significant, unpaired t -test. n =5. Full size image ID4 expression marks a subset of BLBC with poorer prognosis As the factors controlling luminal commitment, such as Brca1 and Elf5 also have well-characterized roles in breast cancer aetiology [29] , [39] , [40] , we next looked at the role ID4 may play in breast cancer. ID4 protein expression in a discovery cohort of 74 breast cancers was largely restricted to ER-negative cases, where it displayed a bimodal pattern of either no staining or strong staining in a majority of cells as seen in 46% of cases ( Fig. 5a,b ). ID4 mRNA followed a similar pattern of expression within the Cancer Genome Atlas (TCGA) data set [41] , with the highest expression in the normal samples and a wide range of ID4 expression observed in the BLBC subtype based on PAM50 classification ( Supplementary Fig. 7a ). To test whether ID4 is important to the biology of ID4 + BLBCs, we knocked down ID4 expression in the MDA-MB-468 BLBC cell line model. Two independent shRNA constructs targeting ID4 significantly reduced proliferation in vitro ( P <0.0001, two-way ANOVA, n =3) ( Fig. 5c ). In addition, ID4 knockdown markedly reduced the growth of MDA-MB-468 xenografts in vivo ( Supplementary Fig. 7b ). It was further confirmed that ID4 knockdown inhibited proliferation of the HCC1806 cell line model of BLBC ( Supplementary Fig. 7c–e ). 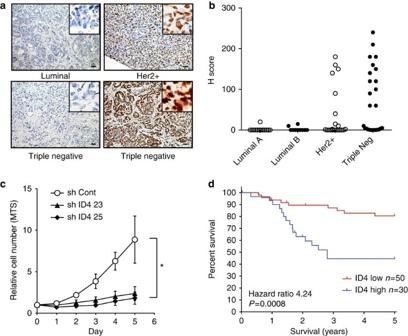Figure 5: ID4 expression, function and clinicopathological correlates in BLBC. (a) Examples of immunohistochemistry staining for ID4 in invasive ductal carcinoma. (b) Quantification of ID4 immunoreactivity in invasive ductal carcinoma by subtype.H-score is a product of staining frequency (%) multiplied by intensity (0–3). (c) Proliferation of MDA-MB-468 cells was measured by the 3-(4,5-dimethylthiazol-2-yl)-5-(3-carboxymethoxyphenyl)-2-(4-sulfophenyl)-2H-tetrazolium, inner salt (MTS) assay following knockdown of ID4 using two independent shRNAs or a control. Graphs represent the mean±s.e.m. (n=3). *P<0.0001, two-way ANOVA. (d) Correlation of ID4 expression with breast cancer-specific survival within a cohort of 80 basal breast cancers, lacking immunoreactivity for ER, PR and Her2, and positive for EGFR, cytokeratin 5/6 or cytokeratin 14. Patients were stratified based on theirH-score with anH-score >10 as ID4 high and anH-score ≤10 as ID4 low.P<0.0008, log-rank test. Figure 5: ID4 expression, function and clinicopathological correlates in BLBC. ( a ) Examples of immunohistochemistry staining for ID4 in invasive ductal carcinoma. ( b ) Quantification of ID4 immunoreactivity in invasive ductal carcinoma by subtype. H -score is a product of staining frequency (%) multiplied by intensity (0–3). ( c ) Proliferation of MDA-MB-468 cells was measured by the 3-(4,5-dimethylthiazol-2-yl)-5-(3-carboxymethoxyphenyl)-2-(4-sulfophenyl)-2H-tetrazolium, inner salt (MTS) assay following knockdown of ID4 using two independent shRNAs or a control. Graphs represent the mean±s.e.m. ( n =3). * P <0.0001, two-way ANOVA. ( d ) Correlation of ID4 expression with breast cancer-specific survival within a cohort of 80 basal breast cancers, lacking immunoreactivity for ER, PR and Her2, and positive for EGFR, cytokeratin 5/6 or cytokeratin 14. Patients were stratified based on their H -score with an H -score >10 as ID4 high and an H -score ≤10 as ID4 low. P <0.0008, log-rank test. Full size image We then asked whether ID4 + BLBCs have a unique clinical phenotype. BLBC is characterized by heterogeneous prognosis, with 30–50% of patients dying of disease within the first 5 years. Immunohistochemistry (IHC) analysis of ID4 expression in a cohort of 80 BLBCs revealed that ID4 + BLBC had a very poor prognosis (hazard ratio 4.24, P <0.0008), with 55% dying of disease within 3 years of diagnosis ( Fig. 5d ). In contrast, only 15% of ID4 − BLBCs died of their disease in this period. Interestingly, the association of ID4 with poor prognosis was independent of tumour grade or proliferative index (Ki67). ID4 mRNA expression also predicted poor prognosis in two independent cohorts of BLBC; 60 BLBCs within the NKI-295 set ( P =0.031) and 285 cases in a compendium of BLBC analysed using the 2014 version of the online analysis tool KM-Plotter [42] ( P =0.0029; Supplementary Fig. 7f,g ). Thus ID4 is highly expressed in ~50% of all BLBCs where it associates with very poor prognosis, and controls in vivo and in vitro proliferation of models of this disease. ID4 marks a subset of BLBC resembling MaSCs The luminal progenitor is thought to be the cell of origin for BLBC, based in part on the observation that the average transcriptome of BLBC most resembles the transcriptome of the luminal progenitor [29] . Given our earlier finding that ID4 marks a MaSC, we hypothesized that the ID4-positive subset of BLBCs may instead resemble a MaSC. To address this hypothesis, BLBC gene expression in the TCGA cohort was stratified based on the top and bottom quartile of ID4 expression and differential gene expression using Limma analysis conducted within these two groups. Six hundred and seventy-one genes were differentially expressed ( q <0.05) between these groups ( Supplementary Data 2 ). ID4 hi BLBCs were enriched for expression of many genes characteristic of adult MaSC and/or fetal murine MaSCs; Itgb1 (1.6-fold), Itga6 (1.9-fold), Sfrp1 (4.9-fold), Wif1 (4.0-fold), Foxc1 (twofold) and Sox10 (fMaSC, 3.9-fold). Strikingly, the contractile actin Actg2 , previously identified as the most highly differentially expressed adult mammary basal/stem cell marker by two independent studies [16] , [43] , was elevated 3.5-fold in ID4 hi BLBCs. Two other myoepithelial contractile actins were upregulated, Acta1 (5.9-fold) and Acta2 (1.7-fold). To systematically address whether ID4 hi BLBC possessed a stem-like gene expression signature, we took two informatic approaches. In the first, we used gene-set enrichment analysis (GSEA) to compare the signature of ID4 hi BLBC with 4,722 curated gene sets within the C2 collection of the Molecular Signatures Database. A large number of gene sets were significantly associated with the ID4 hi BLBC signature, ranked by their normalized enrichment score. These included a number of gene sets associated with breast cancer and tissue stem cells. Interestingly, the 5th most enriched set was the MaSC signature conserved between human and mouse [16] , with a very strong normalized enrichment score of 3.01 ( Fig. 6a,b ). In contrast, the mammary luminal progenitor signature showed no statistically significantly overlap with the ID4 hi BLBC signature. In the second approach, we calculated signature expression scores (SESs) for the MaSC signature in each molecular subtype of breast cancer (as described in Lim et al . [29] ), in addition to the ID4 hi and ID4 lo BLBC subsets. ID4 hi BLBC had a significantly stronger association with the MaSC signature than either the total BLBC set or the ID4 lo BLBC subset ( Fig. 6c ). ‘Claudin low’ breast cancers are a molecular class of triple-negative breast cancers (TNBCs) thought to possess a mesenchymal- and stem-like gene expression signature [44] , [45] and are sometimes grouped with BLBC. However, expression of the definitive claudins 3, 4 and 7 was unchanged between ID4 hi and ID4 lo BLBC ( Supplementary Data 2 ), and analysis of ID4 expression in a panel of TNBC cell lines shows no relationship between ID4 expression and the basal-B mesenchymal-like phenotype [46] , nor with the mesenchymal or mesenchymal stem-like subtypes of TNBC [44] ( Supplementary Fig. 8 ). 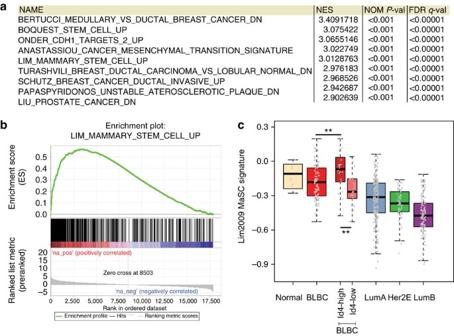Figure 6: Association of the ID4 high basal breast cancer transcriptome with the MaSC signature. (a) Top 10 signatures derived from GSEA analysis of genes differentially expressed between ID4hiand ID4loBLBCs in the TCGA data sets against the Molecular Signatures Database C2 collection of 4,722 gene sets sorted by enrichment (NES). (b) Enrichment analysis of the MaSC signature from Limet al.29compared with the differentially expressed between ID4hiand ID4loBLBCs. (c) MaSC signature expression scores for each subtype and for BLBCs stratified by quartile ID4 expression. **P<0.01, Wilcoxon-Mann-Whitney test. Normal, normal tissue; BLBC, basal-like breast cancer; LumA, luminal A breast cancer; Her2E, Her2-enriched breast cancer; LumB, luminal B breast cancer. Figure 6: Association of the ID4 high basal breast cancer transcriptome with the MaSC signature. ( a ) Top 10 signatures derived from GSEA analysis of genes differentially expressed between ID4 hi and ID4 lo BLBCs in the TCGA data sets against the Molecular Signatures Database C2 collection of 4,722 gene sets sorted by enrichment (NES). ( b ) Enrichment analysis of the MaSC signature from Lim et al . [29] compared with the differentially expressed between ID4 hi and ID4 lo BLBCs. ( c ) MaSC signature expression scores for each subtype and for BLBCs stratified by quartile ID4 expression. ** P <0.01, Wilcoxon-Mann-Whitney test. Normal, normal tissue; BLBC, basal-like breast cancer; LumA, luminal A breast cancer; Her2E, Her2-enriched breast cancer; LumB, luminal B breast cancer. Full size image While the mediators of mammary luminal fate commitment have been extensively described, relatively little is known about the mechanisms controlling MaSCs homeostasis. We now report that Id4 marks a subpopulation of CD24 + CD61 + CD29 hi basal cells that are enriched for the capacity to repopulate a multi-lineage mammary epithelial tree. Furthermore, Id4 deficiency depletes mammary repopulating competency. Id4 hi cells were found distributed throughout the ducts of mature animals and were abundant in TEBs of pubertal mice, which is in stark contrast to Lgr5+ MaSCs recently reported to be concentrated near the nipple and absent from TEBs [47] . These data suggest the existence of multiple stem/progenitor populations differing in anatomical location and development stage. Using single-cell gene expression profiling, we find that Id4 hi cells possess a gene expression signature related to both adult MaSCs [16] and recently identified fMaSCs [36] , suggesting that these two populations may not be mutually exclusive. Id4 + cells also exhibited high expression of Sox9, which is required for MaSC maintenance and which cooperates with Slug to reprogramme luminal epithelium into stem cells [15] . Interestingly, Slug but not Sox9 strongly upregulates ID4 expression [15] , suggesting that Id4, acting downstream of Slug, may cooperate with Sox9 in the maintenance of MaSCs. Although Sox9 was not overexpressed in ID4 hi BLBC, its paralog Sox10 (ref. 48 ), itself a Sox9 target [15] , was highly expressed. Constitutive Id4 overexpression was sufficient to increase the proportion of basal cells in culture and prevented luminal commitment under differentiation conditions. Id4 suppressed expression of key drivers of luminal cell commitment: Brca1, Elf5 and Notch pathway components. Chemical inhibition of Notch activity using the gamma-secretase inhibitor DAPT did not effect Id4 expression but phenocopied Id4 overexpression by downregulating Notch signalling and preventing luminal commitment, suggesting that Id4 controls entry into a luminal fate through Notch inhibition. Interestingly, DAPT treatment, like Id4 overexpression, also downregulated Elf5 expression, revealing a novel regulation of Elf5 downstream of Notch signalling. Loss of Elf5 or Notch signalling is sufficient to prevent luminal differentiation and for accumulation of MaSCs in vivo [5] , [49] , suggesting that regulation of the Notch–Elf5 axis is a critical target of Id4 in preventing luminal commitment. Id4 expression, but not DAPT treatment, inhibited Brca1 expression, indicating that Id4 regulates Brca1 independently of Notch signalling. Dong et al . [23] demonstrated that p38MAPK activity was increased in the mammary epithelium of Id4 −/− mice and that inhibiting p38MAPK could ameliorate some of the proliferative and cell death phenotypes associated with Id4 deficiency. Our data do not contradict these findings; however, they suggest that the increased activity of p38MAPK may be a downstream consequence of abnormal luminal differentiation. Previous studies have shown that p38MAPK activity is increased in luminal MECs during pubertal development and during luminal differentiation in the lung [50] , [51] . BLBCs possess marked molecular and clinical heterogeneity. While 30–50% of patients die of disease within the first 5 years, the remaining patients have very good long-term survival. The discovery of prognostic biomarkers and methods to stratify BLBC into more homogenous subgroups has been difficult. Our data show that ID4 is expressed by ~50% of BLBCs, with these patients having far poorer short-term prognosis than ID4 low BLBC patients, thus ID4 may be an important prognostic factor in this subset of BLBC, especially given the robust IHC test for its expression. While ID4 expression has previously been associated with TNBCs, we uniquely report the ability of ID4 to stratify BLBCs into molecularly or clinically distinct subgroups [52] , [53] , [54] , [55] and validate its prognostic significance in two independent data cohorts. It has previously been suggested that ID4 is a tumour suppressor in breast cancer based on methylation of the ID4 promoter being associated with reduced patient survival [56] , [57] . However, neither of these studies discriminated between molecular or histological subtypes, and BLBC presumably comprised a minority of the samples in these studies. Indeed, evidence from the TCGA breast cancer study demonstrates that luminal B tumours are associated with genome-wide hypermethylation, whereas luminal A tumours are not [26] , leading to the possibility that the observed methylation status of the ID4 promoter was acting as a surrogate to distinguish the poorer prognosis luminal B tumours from the better prognosis luminal A tumours. BLBCs are currently thought to derive from luminal progenitors, based primarily on the accumulation of luminal progenitors in BRCA1 mutation carriers at risk of developing BLBC and the similarity between transcriptional signatures of BLBC and mammary luminal progenitors [29] , [30] . However, these conclusions are based on assumptions of molecular homogeneity within BLBC and that BRCA1-mutant BLBC has the same aetiology as spontaneous BLBC. Our data suggest that BLBCs are heterogeneous in their aetiology, and that the ID4 hi subset possesses a transcriptional signature more similar to the basal cell transcriptome than to luminal progenitors, using two independent informatic approaches. In addition to possessing a stem cell signature, ID4 hi BLBC also expressed high levels of MaSC markers and contractile actins ACTA1, ACTG2 and ACTA2, consistent with a basal/myoepithelial phenotype. There are at least two likely models to explain this observation. The first is that at some time in these cancers a transformed luminal progenitor acquired a stem-like state through dedifferentiation events, as has been recently observed in a mouse model of basal cell carcinoma [58] . The second model is that ID4 hi BLBCs derive from an ID4 hi stem or basal progenitor cell and maintain aspects of the basal phenotype through neoplastic progression, including a stem-like transcriptome and a dependency on ID4 for proliferation. There are other examples of this phenomenon, coined lineage dependency [59] , perhaps best typified by the conserved role for the androgen receptor in prostate development and prostate cancer. Animal models suggest that either model is possible, as mutation of Tp53 and Brca1 in luminal progenitors [30] or basal cells [60] can generate mammary tumours with features of human BLBCs. Interestingly, a majority of murine BLBCs derived from transformation of mammary basal cells express high levels of ID4 ref. 60 as observed in ~50% of clinical BLBC cases. When considered together with our data, these results support the model that ID4 + BLBCs may have an ID4 hi basal cell as their cell of origin. Regardless of the cell from which they derive, ID4 hi BLBC clearly have a unique aetiology and hence may require different clinical management. We predict from the stem-like signature of these tumours an altered therapeutic response compared with ID4 lo disease. Characterization of the gene expression, genomic mutations and therapeutic sensitivity of ID4 hi BLBC may offer insights into molecular dependencies in this class of BLBC and lead to the identification of novel therapeutic opportunities. Mice All experiments involving mice were performed in an specific-pathogen-free animal facility in accordance with the ethical regulations of the Garvan Institute Animal Experimentation Committee. The Id4 GFP/GFP mice were generated as previously described on the C57BL/6 background [31] . These mice were also backcrossed five generations onto the FVB/N strain. Wild-type C57BL/6 and FVB/N mice were also analysed. For xenograft studies, female 8-week-old NOD.CB17-Prkdc scid /Arc mice were used. Mammary gland whole mounts and immunostaining Mammary glands were dissected and whole-mounted at the indicated ages; these were then fixed in 10% neutral-buffered formalin overnight, fat was removed with acetone and the ductal structure was stained with Carmine alum overnight. Glands were then dehydrated through graded alcohols and imaged under methyl salicylate. IHC and IF studies were performed on 4-μm sections of formalin-fixed paraffin-embedded tissue. Antigen retrieval was performed using the DAKO target retrieval reagent 1699 either for 20 min in a boiling waterbath or 1 min in a pressure cooker. The following antibodies were used for IHC and IF analysis, anti-Id4 (1:400, Biocheck, CA, USA), anti-CK8 (1:500, DSHB, IA, USA), anti-p63 (1:100, Novus Biologicals, CO, USA). Envision anti-rabbit reagent (Dako) and DAB (Dako) was used to develop the IHC. Scoring of ID4 expression in human breast cancer samples was scored independently by two individuals based on an H -score, which is derived by multiplying the staining intensity (0–3) with the percentage of epithelial cells with positive nuclear staining. MEC preparations MECs were prepared from freshly obtained 3rd–5th mammary glands pooled from 4–10 female 12-week-old FVB/N mice. Mammary glands were mechanically disrupted with razor blades and then collagenase digested (Collagenase blend type L, 1 mg ml −1 , Sigma). Epithelial cells were enriched by two rounds of differential centrifugation, then the mammary organoinds were further digested with 0.05% trypsin (Invitrogen) followed by Dispase (Stem Cell Technologies). Cells were passed through a 40-μm cell strainer and then resuspended as a single-cell suspension in FACS buffer (PBS 2% fetal bovine serum (FBS) 2% Hepes). Flow cytometry and FACS Single-cell suspensions of primary mouse MECs were incubated with anti-CD16/CD32 antibody (1:200 BD Biosciences) in FACS buffer to block nonspecific antibody binding. Cells were then pelleted and resuspended in FACS buffer containing the following lineage markers: anti-CD31-biotin (1:40 BD Biosciences, Clone: 390), anti-CD45-biotin (1:100 BD Biosciences, Clone:30-F11), anti-TER119-biotin (1:80 BD Biosciences, Clone: TER119), and anti-BP- biotin (1:50 eBiosciences, Clone: 6C3) for 20 min on ice. Cells were then pelleted and resuspended in FACS buffer containing streptavidin-APC-Cy7 (1:400 BD Biosciences) and the following epithelial stem cell markers anti-CD24-PE-Cy7 (1:400, BD Biosciences, Clone: M1/69), anti-CD29-Pacific Blue (1:100 Biolegend (San Diego, CA, USA), Clone: HMβ1-1) and anti-CD61-APC (1:100 Invitrogen, Clone: HMβ1-1), and incubated for 20 min on ice. Cells were then washed twice in FACS buffer before being resuspended in FACS buffer containing DAPI (1:1,000 Invitrogen). Flow cytometry was then performed on a BD LSRII SORP flow cytometer using BD FACSDIVA software, and the results were analysed using Flowjo software (Treestar). Sorting was performed on a BD Influx cell sorter using BD FACSorter software. Mammary transplants Single-cell suspensions of primary mouse MECs were prepared as described above, were resuspended at limiting dilutions in PBS containing magnesium and calcium salts (Gibco/Life Technologies) and then injected into the cleared 4th mammary gland of 3-week-old female FVB/N recipient mice in a 10-μl volume using a Hamilton syringe (Reno, NV, USA). Test and control MECs were injected into contralateral 4th mammary glands. Normal outgrowths were allowed to form for 8 weeks before the glands were harvested and anaylsed by whole-mount histology. Limiting dilution calculations Limiting dilution analysis of MaSC frequency were conducted using the ELDA web interface ( http://bioinf.wehi.edu.au/software/elda/ ) [61] . Cell lines The mouse MEC cell line Comma-Dβ was a gift from Joseph Jeffery (University of Massachusetts, Amherst, MA, USA). Comma-Dβ cells were maintained in DMEM/F12 media (Gibco, Grand Island, NY, USA), supplemented with 2% FBS (Thermo-Scientific), 10 mM HEPES (Gibco), 5 ml penicillin/streptomycin (Gibco), 0.25% insulin (Novo Nordisk, Bagsvaerd, Denmark) and 5 ng ml −1 murine epidermal growth factor (mEGF) (Sigma). MDA-MB-468 cells were obtained from the American Type Culture Collection and maintained in RPMI 1640 media (Gibco), supplemented with 10% FBS (Thermo-Scientific), 20 mM HEPES (Gibco) and 0.25% insulin (Novo Nordisk). HCC1806 cells were obtained from the American Type Culture Collection and maintained in RPMI 1640 media (Gibco), supplemented with 10% FBS (Thermo-Scientific), 20 mM HEPES (Gibco) and 1 mM sodium pyruvate (Gibco). Retroviral transduction of Comma-Dβ cells Comma-Dβ cells (1.1 × 10 5 ) were seeded into a six-well plate. After 16–24 h, the cells were infected with pMSCV-Id4-DSred or pMSCV-DSred retrovirus diluted 1:10 in Comma-Dβ media with 8 μg ml −1 polybrene. After 24 h the media was changed. DSred-positive cells were then FACS enriched using the BD FACSAria fluorescence-activated cell sorter and BD FACSDIVA software. Lentiviral transduction of Comma-Dβ, MDA-MB-468 and HCC1806 cells Cells were seeded into a six-well plate. After 16–24 h, the cells were infected with lentiviruses expressing shRNA constructs diluted 1:10–1:50 into media with 8 μg ml −1 polybrene. After 24 h the media on the cells was replaced with fresh media. Infection efficiency was determined by fluorescence microscopy on cells infected with a control lentivirus expressing EGFP (pLV4301). Lentiviral SMARTchoice Inducible shRNA against Id4 and an irrelevant control were purchased from Dharmacon. HCC1806 cells were infected with virus at a 1:60 dilution with 8 μg ml −1 polybrene and selected with 1 μg ml −1 puromycin for 4 days. Cells were treated at time of seeding with doxycyclin at 1 μg ml −1 , and the cell proliferation assay started once cells had adhered (6 h post seeding) and continued for 94 h. Comma-Dβ in vitro differentiation Comma-Dβ cells were seeded at 0.8 × 10 5 cells per well (or for acute lentiviral knockdown studies at 1.1 × 10 5 as the infection process slowed the growth of the cells) into six-well plates; 72 h later, the media was removed and the cells were washed once with PBS and then media without mEGF was added to the cells. After 24 h (day 0 of the assay), the media was replaced with mEGF-free Comma-Dβ media containing 0.5 μg ml −1 prolactin (Sigma) and 1 nM dexamethasone (Sigma) or fresh mEGF-free media as a control. Media was replaced daily with fresh media containing prolactin and dexamethasone. RNA and protein lysates were collected at day 0, day 2 and day 4. Single-cell analysis was done on cells at the day-2 time point. For the DAPT experiments, 4 μM of DAPT γ-secretase inhibitor (Sigma) or dimethylsulphoxide control was added to the mEGF-free media on D0. Media was replaced daily with fresh media containing DAPT or dimethylsulphoxide. Assay for cell proliferation MDA-MB-468 cells were seeded at 3.2 × 10 3 per well in a 96-well flat-bottomed plate. On days 0, 1, 2, 3, 4 and 5, following seeding, 20 μl 3-(4,5-dimethylthiazol-2-yl)-5-(3-carboxymethoxyphenyl)-2-(4-sulfophenyl)-2H-tetrazolium, inner salt (MTS, Promega) was added to each well and incubated at 37 °C in 5% CO 2 and 95% air in a tissue culture incubator for 3 h before measuring absorbance at 490 nm using a FLUOstar Optima plate reader with Optima software (BMG LabTech). On day 0, cells were allowed to adhere for 4 h before adding MTS solution. An average of the six replicate wells was taken and the blank absorbance value was subtracted. All samples were normalized to the day-0 absorbance of the same cell line and short hairpin construct; that is, on day 4, shID4 23 was normalized to the day-0 shID4 23 absorbance reading. Relative cell proliferation of HCC1806 cells was calculated using IncuCyte ZOOM live cell imaging (zoom40061 Essen BioScience). Xenografts Surgery was performed as previously described. A total of 1 × 10 6 cells were transplanted in 10 μl sterile PBS containing magnesium and calcium salts. Cells were injected into the fourth thoracic mammary fat pad of 5-week-old female NOD.CB17-Prkdc scid /Arc mice. Five mice per group (ID4 knockdown and control cell transplants). Tumour volume was measured twice weekly by a technician blinded to the identity of mice. Tumours were harvested when control tumours reached 10 mm by the longest diameter. Western blotting Protein lysates (5–20 μg) were prepared with 4 × loading buffer (Invitrogen) and sample reducing agent (Invitrogen), denatured by heating to 70 °C for 10 min and loaded onto 4–12% bis/tris gels (Invitrogen). Gels were run at 200 V for ~40 min using MES running buffer (Invitrogen). Proteins from the gels were then transferred to Hybond ECL nitrocellulose membranes (Amersham Biosciences, Germany) using the Invitrogen western blotting module and transfer buffer for 1–1.5 h at 30 V. Membranes were then rinsed in TBST and blocked for 1 h at room temperature (or overnight at 4 °C) in either TBST 5% skim milk powder (or TBST 2% BSA for the anti-milk and anti-phospho protein western blots). Antibodies used for western blotting were anti-Id4 (1:25,000, Biocheck), anti-Milk proteins (1:10,000, Accurate Chemical & Scientific Corp), anti-p38 MAPK (1:1,000, Cell Signalling), anti-phospho-p38 MAPK (1:1,000 Cell Signalling) and anti-β−Actin (1:100,000, Sigma). Western blot bands were visualized using Western lightning Plus ECL reagent (Perkin Elmer, Waltham, MA, USA) and Fuji SuperRX film (Tokyo, Japan). Quantitative RT–PCR RNA was extracted from cells using either Trizol (Ambion/Life Technologies) or the RNAeasy Minikit (Qiagen) following the manufacturer’s instructions. RNA was eluted or resuspended in nuclease-free water (Promega). RNA was extracted from mammary glands using the RNAeasy Minikit as follows. 20–30 mg of snap-frozen mammary gland pieces were ground in microcentrifuge tubes on dry ice using a 1.5-ml pellet pestle (Lomb Scientific/Thermo-Scientific) for roughly 10 s until all large pieces are broken up. Six hundred μl of buffer RLT was added and then the sample was sonicated on ice for a total of 20 s with 2-s pulses and 0.5-s pauses. RNA extraction was then continued as per the Qiagen RNAeasy minikit protocol. Complementary DNA (cDNA) was synthesized from 0.5–1 μg of RNA using the Superscript III RT–PCR kit (Invitrogen) using oligo-dT primers and following the manufacturer’s instructions. TaqMan probes (Applied Biosystems/Life Technologies) were used to analyse mRNA expression levels as per manufactures specifications ( Table 2 ) using an ABI PRISM 7900 HT machine. Table 2 QRT–PCR assays used for gene expression studies. Full size table Acquisition of TCGA data Clinical and molecular annotation of samples was obtained from the marker TCGA BRCA publication ( Supplementary Table 1 in TCGA Nature 2012, PMID: 23000897). Agilent mRNA expression microarray data (level 3) was obtained from the TCGA data portal in January 2012. The microarray data consisted of 8 normal-like, 98 basal-like, 58 Her2-enriched, 231 luminal A and 127 luminal B tumours. Two methods were used for replacing missing expression values: for GSEA analysis missing values were imputed and replaced using the k -nearest-neighbour approach, with k =10; for SES analysis missing values were replaced with the median gene expression value of 0. The samples classified as PAM50 basal-like were stratified on expression of ID4, and the top 25% (ID4 hi ) and bottom 25% (ID4 lo ) expressing samples were selected (see Supplementary Data 3 for a list of the stratified patient sample barcodes and ID4 expression level). Analysis of TCGA expression data Differential gene expression between the ID4 hi and ID4 lo basal-like patient groups was assessed for each gene using an empirical Bayes, moderated t -statistic implemented in Limma [62] via the limmaGP tool in GenePattern. GSEA [63] was run with the GenePattern tool GSEApreranked using a ranked list of the Limma moderated t -statistics against the curated gene sets from version 4.0 of the Molecular Signatures Database [63] . The minimum and maximum gene-set sizes used were 15 and 500, respectively, with 1,000 permutations performed. All analyses were performed using GenePattern [64] software modules, which are available at http://pwbc.garvan.unsw.edu.au/gp/ . Subtype expression signature analysis Subtype SES analysis was carried out using the TCGA Agilent mRNA microarray expression data and the mammary cell-lineage-specific gene sets as described in ref. 29 . Specifically, an expression signature score was calculated for each of the 522 samples identified from the TCGA Agilent mRNA microarray expression data set. A higher score indicates that the breast cancer sample is more positively correlated with the mammary cell-lineage gene signature. Subtype expression signature scores, s , were calculated as follows, where the sum is over all genes, g , in the mammary cell-lineage-derived expression signature gene sets, x g is the log-fold change for that gene in the cell lineage signature and y g is the log2 expression for the same gene in the TCGA sample. Non-matching gene symbols were discarded and for each gene only the probe with highest expression level was used. The TCGA samples were then stratified into PAM50-predicted molecular subtypes and the ID4 hi - and ID4 lo -expressing basal-like subsets (as described above). P values were calculated between each sample set using the Wilcoxon–Mann–Whitney test. Analysis of ID4 protein expression in breast cancer subtypes Samples were obtained from the Australian Breast Cancer Tissue Bank and had been classified as luminal A, luminal B, Her2-positive or triple negative based on expression of ER, PR and Her2. A separate BLBC cohort used for survival analysis was classified based on lack of ER, PR and Her2 expression but positive staining for EGFR, cytokeratin 5/6 or cytokeratin 14, and stained for Id4 using a rabbit monoclonal antibody (Biocheck). IHC was scored by a trained pathologist blinded to the identity of specimens. The H -score was determined by multiplying the staining intensity (0–3) with the percentage of positive nuclei. Analysis of the NKI-295 data set Data were taken from array profiling of the NKI-295 breast cancer cohort [65] , and basal breast cancers were identified using a single sample predictor [66] . Samples were allocated into ID4 high versus low using mixture modelling and the association with overall survival analysed. Single-cell analysis Comma-Dβ cells were seeded at 8 × 10 4 cells per well into six-well plates, 96 h later (day 0) the media was removed, cells were washed twice with PBS and media was replaced without mEGF. Day 2, cells were collected in a single-cell suspension of a concentration of 250K ml −1 in native medium. Using the C 1 Single-Cell Auto Prep System (Fluidigm) the cells were loaded onto a C 1 Single-Cell Auto Prep Integrated Fluidics Circuit (IFC) and captured and stained for viability with the LIVE/DEAD Cell Viability/Cytotoxicity Kit (Invitrogen). Subsequent cell lysis, reverse transcription and 18 cycles of preamplification using a pooled primer mix of all target gene F/R primers was performed on the microfluidic device. Tube control samples of 1,000 cells were processed off-chip in parallel as positive controls. Amplified cDNA libraries from each single cell on the IFC were harvested in 3 μl and diluted in 25 μl of C1 DNA dilution buffer. The diluted cDNA was then mixed with TaqMan Gene Expression MasterMix (Life Technologies) and loading reagents (Fluidigm) and introduced onto a 96.96 gene expression Dynamic Array IFC (Fluidigm) for quantitative (q)RT–PCR analysis. The same TaqMan assays used in the single-cell preamplification were used for qRT–PCR ( Supplementary Data 1 ). Samples and assays were mixed in a 96 × 96-format, amplified and measured for fluorescence using a BioMark HD genetic analysis system (Fluidigm). The two data files were independently loaded into the Fluidigm Real-Time PCR Analysis software (v 4.0.1) and then manually edited to remove any failed reactions. As the two data sets had been run on separate chips, a normalization step was required to ensure the data could be combined without bias. This was achieved by performing independent normalization calculations for each cell using the arithmetic mean of the three housekeeping genes ( Gapdh , Hprt and Rplp0 ). Once combined, the Id4 high and low cells were identified by selecting the upper and lower quartiles of the normalized cycle threshold (CT) values and labelled as such. The edited file was then analysed using the SINGuLAR software (v 2.0.2, ( http://www.fluidigm.com/singular-analysis-toolset.html ), whereby outlier samples were identified, before principal component analysis (PCA), ANOVA and unsupervised clustering analysis were performed. How to cite this article: Junankar, S. et al . ID4 controls mammary stem cells and marks breast cancers with a stem cell-like phenotype. Nat. Commun. 6:6548 doi: 10.1038/ncomms7548 (2015).